Repeating microearthquake sequences interact predominantly through postseismic slip Studying small repeating earthquakes enables better understanding of fault physics and characterization of fault friction properties. Some of the nearby repeating sequences appear to interact, such as the ‘San Francisco’ and ‘Los Angeles’ repeaters on the creeping section of the San Andreas Fault. It is typically assumed that such interactions are induced by static stress changes due to coseismic slip. Here we present a study of the interaction of repeating earthquakes in the framework of rate-and-state fault models using state-of-the-art simulation methods that reproduce both realistic seismic events and long-term earthquake sequences. Our simulations enable comparison among several types of stress transfer that occur between the repeating events. Our major finding is that postseismic creep dominates the interaction, with earthquake triggering occurring at distances much larger than typically assumed. Our results open a possibility of using interaction of repeating sequences to constrain friction properties of creeping segments. Interaction of earthquakes, which is quite important for uncovering fault physics and quantifying seismic hazard, has been widely studied but, owing to large variations in where and how it occurs, the governing physical mechanisms are still unclear [1] , [2] . Advancing the time of instability by a favourable static stress change due to coseismic slip is most commonly used in modelling aftershock sequences [3] , [4] . However, triggering can also be found in areas of unfavourable static stress changes and at distances beyond the reach of significant static stress changes. Other proposed interaction mechanisms include dynamic stress changes due to seismic waves [5] , [6] , [7] , increased stress loading rate due to aseismic slip [8] , [9] or relaxation of the viscoelastic lower crust [10] , [11] , pore fluid motion and induced variations in fault strength [12] , and evolution of viscoelastic damage rheology due to sudden increase in strain [13] . Earthquake triggering may involve a combination of several mechanisms. Here we aim to quantify the relative importance of several triggering mechanisms using numerical simulations of small repeating earthquakes. Owing to their short recurrence times and known locations, small repeating earthquakes are highly suited for studies of earthquake physics [14] , [15] , [16] , [17] and, in particular, earthquake interaction [18] . For example, the ‘San Francisco’ (SF) and ‘Los Angeles’ (LA) repeating sequences in Parkfield, California, which are among the primary targets of the San Andreas Fault Observatory at Depth drilling project, have a lateral separation of <70 m [16] , [17] . The LA events tend to occur shortly after the SF events, suggesting a triggering effect [16] . We find that static stress changes due to postseismic slip dominate the interaction of repeating earthquakes on creeping segments. The associated propagating stress front causes the interaction to extend much farther—to 4–7 rupture diameters—than would be predicted based on static stress changes from coseismic slip alone. Conversely, for the same separation distance, the interaction would be much stronger than predicted based on stress changes due to coseismic slip. These findings motivate using interaction of small repeating earthquakes to constrain the friction properties of the surrounding creeping regions. Simulations of repeating earthquake sequences We study interaction of repeating earthquakes in the framework of rate-and-state fault models [19] . In the models, repeating earthquakes occur on velocity-weakening (VW) patches embedded into a larger velocity-strengthening (VS) fault area ( Fig. 1a ). Such models have been shown to reproduce the behaviour of isolated repeating earthquake sequences, in particular the scaling of their moment versus recurrence time and the response to accelerated postseismic creep [20] , [21] . Outside the VS region, slow slip with the long-term fault slip rate is imposed, as would be appropriate for the larger creeping segment. Our simulations produce realistic fault responses, including stick-slip behaviour of the patches with aseismic nucleation processes, seismic events with slip rates of the order of 1 m s −1 and postseismic slip ( Fig. 1 and Supplementary Fig. 1 ). This is due to the state-of-the-art simulation methodology that combines slow tectonic-like fault creep with all wave-induced effects during seismic events. The modelling allows us to compare effects of static stress changes due to coseismic and postseismic slip, as well as dynamic stress changes due to seismic waves. 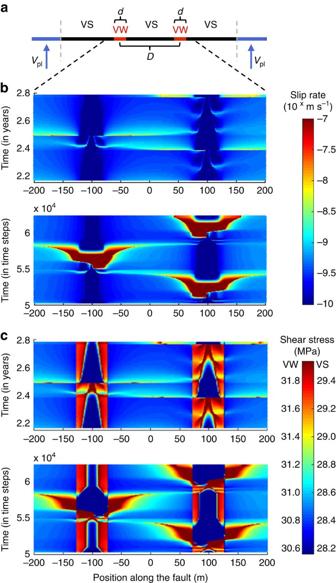Figure 1: Interaction of two repeating earthquake sequences in a rate-and-state fault model. (a) Schematics of the model in which a one-dimensional fault is embedded into elastic medium and loaded with slow, tectonic slip rate (Vpl)of 23 mm per year. The fault contains two seismogenic VW patches surrounded with VS regions.Dis the separation distance between the centre of the two VW patches anddis the diameter of each patch. (b,c) Evolution of slip rate (b) and shear stress (c) on the fault with the simulated time (top) and as functions of variable time step (bottom). The colour scales are chosen to emphasize the slip rates and stress values relevant to postseismic effects. Seismic events start at an edge of a VW patch and spread through the patch, penetrating into and eventually stopping in the surrounding VS regions. The resulting postseismic creeping fronts (PCFs) are clearly observed travelling from one patch to the other. The PCF from the right patch advances the seismic event on the left patch. The PCF from the left patch triggers some aseismic slip on the right patch, but without changing the timing of the event appreciably. The time-dependent evolution of the slip rate is also shown inSupplementary Movie 1. The formulation of the model and its parameters are summarized in ‘Methods.’ Figure 1: Interaction of two repeating earthquake sequences in a rate-and-state fault model. ( a ) Schematics of the model in which a one-dimensional fault is embedded into elastic medium and loaded with slow, tectonic slip rate ( V pl )of 23 mm per year. The fault contains two seismogenic VW patches surrounded with VS regions. D is the separation distance between the centre of the two VW patches and d is the diameter of each patch. ( b , c ) Evolution of slip rate ( b ) and shear stress ( c ) on the fault with the simulated time (top) and as functions of variable time step (bottom). The colour scales are chosen to emphasize the slip rates and stress values relevant to postseismic effects. Seismic events start at an edge of a VW patch and spread through the patch, penetrating into and eventually stopping in the surrounding VS regions. The resulting postseismic creeping fronts (PCFs) are clearly observed travelling from one patch to the other. The PCF from the right patch advances the seismic event on the left patch. The PCF from the left patch triggers some aseismic slip on the right patch, but without changing the timing of the event appreciably. The time-dependent evolution of the slip rate is also shown in Supplementary Movie 1 . Full size image Strong earthquake interaction To study earthquake interaction, it is important to set up a quantitative measure of the interaction. Two repeating sequences are typically considered interactive if the events of one of them occur within a short time of the other. For instance, the inter-event time between the LA and SF repeating sequences is usually <24 h (ref. 16 ). To enable the quantification of interaction in our model, we assign the initial conditions on the fault such that the two patches, if not interacting, would produce earthquakes as far in time from each other as possible, or half of their recurrence interval T r apart. This is accomplished by first conducting a single-patch calculation and recording the conditions on the patch when it is 0.4 T r or 0.9 T r after a seismic event ( Supplementary Fig. 2 ). We then assign these slip rate, stress and state conditions as the initial ones in the two-patch simulation ( Supplementary Fig. 3 ). If the patches do not interact, then one of them is expected to produce an earthquake in 0.1 T r and the other one in 0.6 T r , as happens in the single-patch calculation, making the events 0.5 T r apart. Indeed, we find that when the distance D between the two patches is large enough ( D =15 d , where d is the patch diameter), each of them behaves as an isolated repeating sequence, with events on the two patches separated by 0.5 T r ( Fig. 2 and Supplementary Fig. 4a ). If the patches interact, the events on the patches occur closer in time. 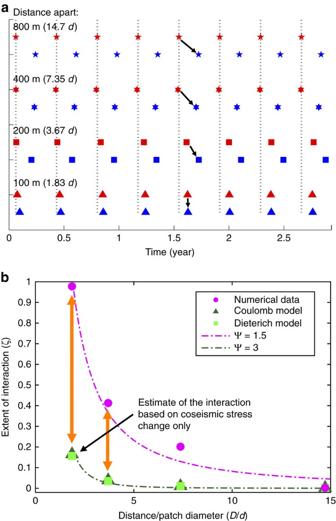Figure 2: Exploring the extent of interaction between the two repeating earthquake sequences. (a) Dependence of the interaction on the distance between the patches. Red and blue markers represent the occurrence of seismic events on the two VW patches. Patches in the simulation withD=15drupture with the expected interevent time of half of the single-patch recurrence time, and hence they are non-interacting. The inter-event times decrease significantly as the distance between the two VW patches reduces. Dashed lines mark the recurrence interval for the non-interacting case. (b) Extent of interaction in our simulations (circles) plotted against separation distanceD/d. Estimates of the interaction based on the coseismic stress changes only for the Coulomb and Dieterich models are shown as triangles and squares, respectively. Orange arrows indicate the inferred effect of postseismic creep which clearly dominates. Dashed lines show the fit of the results to a power lawζ=(D/d)−Ψ. The difference ζ between the simulated inter-event time Δ T sim and the non-interacting inter-event time 0.5 T r , normalized by 0.5 T r , can serve as the measure of the degree of interaction: Figure 2: Exploring the extent of interaction between the two repeating earthquake sequences. ( a ) Dependence of the interaction on the distance between the patches. Red and blue markers represent the occurrence of seismic events on the two VW patches. Patches in the simulation with D =15 d rupture with the expected interevent time of half of the single-patch recurrence time, and hence they are non-interacting. The inter-event times decrease significantly as the distance between the two VW patches reduces. Dashed lines mark the recurrence interval for the non-interacting case. ( b ) Extent of interaction in our simulations (circles) plotted against separation distance D / d . Estimates of the interaction based on the coseismic stress changes only for the Coulomb and Dieterich models are shown as triangles and squares, respectively. Orange arrows indicate the inferred effect of postseismic creep which clearly dominates. Dashed lines show the fit of the results to a power law ζ =( D / d ) −Ψ . Full size image As expected, based on intuition and prior studies [3] , [4] , the two seismogenic patches behave independently when they are far apart and rupture together if they are right next to each other. In the intermediate range of distances, ruptures on the two patches cluster in time ( Fig. 2a ). As the distance D between patches decreases, we start to observe interaction, with the inter-event time Δ T sim decreasing from 0.5 T r =2.3 months for D =14.7 d to 1.3 days for D =1.83 d . Hence, the extent of the interaction ζ increases from 0 (no interaction) to nearly 1 ( Fig. 2b ). Importantly, there is appreciable interaction at distances as large as 4 d ( ζ =0.4) and even some interaction at distances of 7 d ( ζ =0.2). For a larger VW patch, interaction extends even farther, with ζ =0.3 even at distances D =15 d ( Supplementary Fig. 5 ). These results are surprising given the interaction distances of 1 to 2 rupture diameters typical for static stress changes. Our simulations reveal that in addition to the static stress increases caused by the coseismic slip of one patch on the other patch, interaction also occurs through accelerated postseismic slip between the two patches. In fact, for a wide range of model parameters, we find the accelerated aseismic slip to be the determining factor in triggering seismic events nearby. To compare the magnitude of different stress changes potentially contributing to triggering, let us consider the shear stress experienced by the centre of each VW patch, focusing on the time between two events ( Fig. 3 ). As patch 1 ruptures (red near-vertical line in Fig. 3 ), it produces several types of stress changes on patch 2 (blue line in Fig. 3 ). First, dynamic wave-mediated stress changes occur, but they do not seem to have any appreciable effect in our models, consistent with prior studies in rate-and-state models [22] , [23] . Right after the end of the seismic event, patch 2 gets a static stress increase due to the coseismic slip on patch 1, appearing as a relatively small vertical jump of ∼ 0.1 MPa at t =2.39 yr marked as (I) in Fig. 3 . The static stress increase is experienced by other points on the fault as well and it causes accelerated aseismic slip in the VS area known as afterslip. This accelerated aseismic slip has two kinds of effects on patch 2. First, the stress of patch 2 starts to increase at a faster rate due to the response of the VS area adjacent to patch 2, from 2.39 to 2.415 yr in Fig. 3 , marked as (II). Second, the travelling postseismic front, visible in Fig. 1b,c as a yellow to light blue area spreading from one patch to the other, brings with it even larger stressing rate increases, making this last effect dominant in our model ( Fig. 3 , from 2.415 to 2.43 yr, marked as (III)). The shear stress loading slows down after the passage of the postseismic stress front (from 2.43 yr onward) but still remains higher than the pre-seismic rate. Shortly before 2.5 yr, patch 2 responds dynamically. In this simulation, the two VW patches are ∼ 3.7 d apart and ζ =0.54. At shorter distances between patches, patch 2 typically ruptures even sooner after the creeping front arrives. 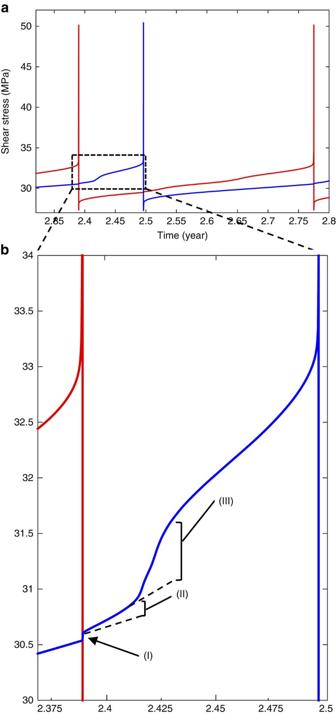Figure 3: Different types of stress changes induced on the triggered VW patch. (a) Shear stress as a function of time in the centre of the triggering patch (red line) and triggered patch (blue line). (b) Zoom into the dashed rectangle of the top panel shows three types of stress increases in the triggered patch: (I) direct static stress change due to coseismic slip on the other patch; (II) stress change due to elevated stressing rate in the VS region adjacent to the triggered patch; (III) stress change due to propagating postseismic creep. Postseismic stress changes (II) and (III) are clearly much larger than the stress change (I) due to coseismic slip only. Figure 3: Different types of stress changes induced on the triggered VW patch. ( a ) Shear stress as a function of time in the centre of the triggering patch (red line) and triggered patch (blue line). ( b ) Zoom into the dashed rectangle of the top panel shows three types of stress increases in the triggered patch: (I) direct static stress change due to coseismic slip on the other patch; (II) stress change due to elevated stressing rate in the VS region adjacent to the triggered patch; (III) stress change due to propagating postseismic creep. Postseismic stress changes (II) and (III) are clearly much larger than the stress change (I) due to coseismic slip only. Full size image The interaction between patches produces other more subtle but interesting effects. Compared with the non-interacting case, the recurrence interval of VW patches is slightly lengthened for cases with shorter separation distances ( D =3.7 d and 1.83 d ; Fig. 2a and Supplementary Fig. 4b ). However, the recurrence interval getting longer in two-patch simulations is not a universal effect; in some simulations, the recurrence interval of the VW patches in the two-patch simulation becomes shorter than that in the one-patch simulation ( Supplementary Fig. 6 ). The difference between the recurrence intervals in the single-patch and two-patch simulations probably results from the combination of two factors: the response of the patches to induced stress changes in the two-patch simulations and the difference in seismic events that occur on the patches in the two simulations, as described in the Discussion section. Dominance of postseismic stress change How can we compare what appears to be, based on the stress changes ( Fig. 3 ), the dominating effect of the postseismic slip with the effect of the directly induced static stress changed due to coseismic slip (with the latter being the typical explanation for earthquake interaction)? We can estimate the time advance of the triggered earthquake due to the static stress increase caused by coseismic slip alone; the difference between that and the simulated time advance should be due to the postseismic effects. The time advance due to the coseismic slip can be estimated in two ways, based on the Coulomb failure model [24] and Dieterich rate-and-state model [25] . The Coulomb model has a simple failure criterion of shear stress τ reaching a critical friction threshold of μ ( σ − p )+ S , where σ is the normal traction (positive in compression), p is the pore fluid pressure, μ is the friction coefficient and S is the cohesion [24] . Hence, the fault is brought closer to failure for positive changes of Δ CFS =Δ τ − μ (Δ σ −Δ p ), which correspond to the time advance of , where is the background stressing rate. In our models, Δ CFS =Δ τ . In the Dieterich model, the time to instability T for a nucleation site with slip velocity V is analytically evaluated based on the spring-slider approximation of elastic interactions and an assumption on the state variable evolution [25] : where is the effective normal stress, a , b and L are rate-and-state parameters (see Methods) and k is the spring stiffness (and hence the effective stiffness of the nucleation site). A positive step in shear stress (Δ τ ) increases slip rate V to V new =exp[Δ τ /( a ( σ − p ))], thus shortening the time to the next rupture. The difference Δ T DM = T ( V )− T ( V new ) between the two times to instability constitutes the time advance due to Δ τ . From our simulations, we can obtain the interseismic stress loading rate and positive shear stress step Δ τ occurring on the triggered patch due to coseismic slip on the other patch. The stiffness of the nucleation patch can be approximated [22] as k = ηG / h nucl , where η =2/ π , G is the shear modulus and h * is the nucleation size given by [26] : Hence, we can estimate the corresponding time advances Δ T CM and Δ T DM , which are about an order of magnitude smaller than the simulated time advance ( Fig. 2b ), confirming the dominant effect of the stress changes due to postseismic slip. Our finding that the interaction of earthquakes on creeping segments may be dominated by their postseismic slip opens the possibility of estimating fault friction properties based on modelling the interaction. The postseismic slip depends on the stress drop of the seismic event—which determines the stress increase on the surrounding creeping fault regions—as well as the steady-state velocity strengthening of the creeping region [8] ; the latter effect is demonstrated in Supplementary Fig. 7 . Values of ( a − b ) much larger than the ones estimated in the laboratory impede postseismic slip and remove its triggering effect ( Fig. 4a ). If the stress drops are known, one can determine, through modelling, the range of values of that reproduce observations. 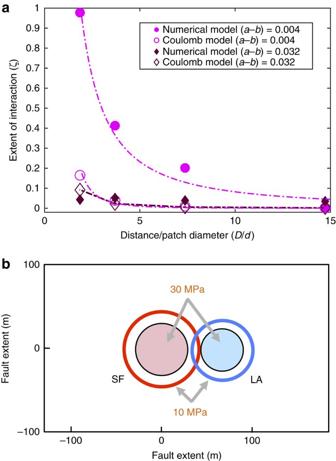Figure 4: Effect of the VS region on the interaction. (a) Comparison of interaction with different friction properties of the VS region: (a−b)VS=0.004 (circles) and 0.032 (diamonds). Filled and empty markers represent our numerical model and Coulomb model, respectively. Postseismic creep (and its effect) is suppressed as (a−b)VSincreases from 0.004 to 0.032. (b) Schematic diagram of the relative location of the SF and LA repeaters based on the study of Zobacket al.17. The extent of the patches for both 10 MPa (empty circles) and 30 MPa (filled circles) stress drops are shown;D/dchanges with different stress drop estimates. For the stress drops of 30 MPa, the repeaters are separated by about 1.4 average patch diameters; the nearly instantaneous triggering observed for these repeaters before 2004 is consistent with our findings and can be used to constrain the VS properties of the creeping region. Figure 4: Effect of the VS region on the interaction. ( a ) Comparison of interaction with different friction properties of the VS region: ( a − b ) VS =0.004 (circles) and 0.032 (diamonds). Filled and empty markers represent our numerical model and Coulomb model, respectively. Postseismic creep (and its effect) is suppressed as ( a − b ) VS increases from 0.004 to 0.032. ( b ) Schematic diagram of the relative location of the SF and LA repeaters based on the study of Zoback et al . [17] . The extent of the patches for both 10 MPa (empty circles) and 30 MPa (filled circles) stress drops are shown; D / d changes with different stress drop estimates. For the stress drops of 30 MPa, the repeaters are separated by about 1.4 average patch diameters; the nearly instantaneous triggering observed for these repeaters before 2004 is consistent with our findings and can be used to constrain the VS properties of the creeping region. Full size image For the LA and SF repeaters on the San Andreas Fault, determining the constraints on friction due to postseismic-slip-dominated interaction would involve first determining which source properties (including stress drop) better fit the available seismic data. Currently, stress estimates for small earthquakes are typically obtained from a widely used relation for a circular crack of radius r with the constant stress drop Δ τ and moment M o : Δ τ =(7 M o )/(16 r 3 ), in which the moment is well constrained and the radius r is determined from the source spectra and its corner frequency based on simplified source models [27] . For the LA and SF sequences, such stress drop estimates are in the range of 10–30 MPa [27] , [28] , [29] , depending on the simplified source model used. If the stress drops of the LA and SF repeaters are indeed ∼ 10 MPa, then, given the inferences of their separation, the patches are large enough to be right next to each other ( Fig. 4b ). In our model, they would essentially rupture in a single dynamic event. If the stress drops are closer to 30 MPa, then the events are separated by about 1.4 diameters of the repeaters (taking the average diameter of the two patches), similar to the shortest inter-patch distance of D =1.83 d considered here. In that case, based on our modelling so far, the interaction should be dominated by postseismic slip and hence by the VS friction properties of the area between the patches. The absence of the LA–SF interaction after the 2004 Mw 6.0 Parkfield earthquake may be due to the increase in the value of between the patches, for example, due to decrease in pore pressure. Determining the realistic source properties of the LA and SF repeaters based on seismic data, as well as constraining the VS properties between the patches based on the interaction would require a targeted three-dimensional modelling of the two repeaters, in which a two-dimensional fault is embedded into a three-dimensional elastic medium, with patches represented as circles, a subject of our ongoing work. It is noteworthy that such much more computationally challenging modelling could not be used in this work, as it would make the longer inter-patch distances D / d =15 considered here computationally intractable in the context of simulating earthquake sequences. The interaction of the two patches in our simulations is influenced by multiple kinds of stress changes received at different times of their interseismic period ( Fig. 3 ); this complexifies the resulting patch behaviour. One such complexity is that the recurrence time of interacting patches may be either shorter or longer than that of identical patches that do not interact. This is due to a combination of two factors. First, after seismic event I on patch 1 triggers a seismic event II on patch 2, the (favourable) stress perturbations from event II reach patch 1 early in its interseismic cycle and such stress perturbations sometimes advance and sometimes delay the nucleation process. The delay can result if the (favourable) stress changes lead to a nucleation-size aseismic transient, relieving stresses in the nucleation zone and delaying the next seismic event [23] . Second, different stress conditions on the patches before a seismic event—due to ongoing stress interactions as well as due to rupture nucleation in a slightly different location within the patch—can cause the resulting seismic slip on the patches to be slightly different, corresponding to different stress drops and hence different required interseismic loading times. The intricate interplay between these interrelated factors needs to be investigated further. It may at least partially explain the irregularity of the observed repeating sequences, which are likely to be continuously perturbed not only by each other, as in the case of the LA and SF repeaters, but also by other seismic events nearby, as well as potential interseismic phenomena such as unsteady creep elsewhere on the fault [30] . To enable the precise quantification of the interaction and quantitative comparison between the effects of various stress changes, we have focused here on the models with the initial conditions that put the two patches half a cycle (0.5 T r ) apart; the results should hold for other initial conditions as well, based on the following consideration. If the first event on patch 1 occurs when patch 2 is closer to failure than half a cycle, then the extent of interaction between patches should be the same or greater than in the half-a-cycle-apart case. If the first event on patch 1 occurs when patch 2 is farther from failure than half a cycle, then that particular event may have smaller or no effect; however, at the time of the next seismic event on patch 2, patch 1 should be closer to failure than half a cycle and the interaction should again be the same or greater than in the half-a-cycle-apart case, but with the patch roles reversed (patch 2 triggering patch 1). This is essentially what our simulations show. For example, for large enough patches ( d =82 m=4.1 h * and 108 m=5.4 h *, where h * is the nucleation size for the VW patches given by (4)), and patch separation distance D =1.83 d , the eventual behaviour is that of seismic events on one patch triggering seismic events on the other patch nearly instantaneously compared with their recurrence interval, for all initial conditions we have explored ( Supplementary Figs 6, 8 and 9 ). This is also true for several cases of initial conditions for smaller patches ( d =40 m=2 h * and 54 m=2.7 h *; Fig. 2 and Supplementary Figs 8 and 9 ). Some initial conditions on smaller patches lead to more complex behaviour, with the two patches initially moving towards such rapid triggering, but then gradually evolving to the long-term state in which the two patches consistently rupture half a cycle (0.5 T r ) apart ( Supplementary Figs 8–10 and Supplementary Table 1 ). It is noteworthy that such a pattern also represents interaction strongly influenced by postseismic slip, not only because substantial triggering is indeed observed at the beginning of the simulations, but also because the long-term behaviour is different from the predictions based on coseismic stress changes only ( Fig. 2b ). According to both Coulomb and Dieterich predictions, coseismic stress changes imposed by a seismic event on patch 1 onto patch 2 should advance the next seismic event on patch 2 by 15–20% ( Fig. 2b ). The fact that this does not happen in the simulations is probably related to the additional influence of the postseismic stress changes. Ultimately, this evolving behaviour is due to the interplay of seismic and substantial aseismic slip—both spontaneous and interaction induced—on such smaller patches, which would be completely aseismic if they were smaller than h * (ref. 20 ). This apparent precise cancellation among all triggering effects will probably disappear in a more realistic three-dimensional model, especially in the presence of spatial heterogeneity in fault friction properties that is likely to exist on natural faults and perturb the regularity of the patch recurrence. It is worthy noting that the patch behaviour is dependent on the ratio of d / h *, because the ratio of aseismic to seismic slip on the patches systematically increases as the patch diameter d decreases to the nucleation size h * (ref. 20 ). The potentially dominant effect of postseismic slip on the interaction of repeating earthquakes demonstrated by our modelling adds to the growing realization of the importance of aseismic slip in earthquake source processes, even in phenomena long thought to be dominated by seismic slip. This includes the suggestion that aftershock sequences may be at least partially controlled by aseismic slip [8] as well as with the observations that fluid injection into fault zones may trigger aseismic slip which, in turn, at least helps to trigger microseismicity [31] , [32] . Our findings motivate further development of earthquake source models that faithfully reproduce the interaction between seismic and aseismic fault slip, such as realistic source models of the Parkfield repeaters constrained by the wealth of available data [17] . The rate-and-state fault model Our numerical simulations are based on a two-dimensional elastodynamic model of a one-dimensional fault embedded into an elastodynamic medium. The fault is governed by laboratory-derived rate-and-state friction laws, which have been quite successful in reproducing a number of earthquake phenomena [33] . The shear strength is given by: where τ f is the shear strength of the fault, is the effective normal stress, f is the friction coefficient, f o is the reference friction coefficient at the reference slip velocity V o , a and b are rate-and-state parameters, V is the slip velocity and L the characteristic slip for the evolution of the state variable θ . In steady state, when V is constant, one gets θ = L / V and the resulting shear stress ( τ ss ) is: Hence, an interface with a − b <0 has VW friction, whereas a − b >0 corresponds to VS friction. On the fault, two VW patches are surrounded by VS regions ( Fig. 1a ); outside, the long-term slip rate is imposed. Parameters of the model are listed in Table 1 ; the values of a and b in the VS region as well as the patch diameter are varied in some simulations as specified when the simulations are discussed. Stresses, slips and slip rates within the VW and VS regions are computed by equating the fault shear stress given by elastodynamic relations with the fault strength given by the friction law (4–5) [34] . We make the size of the friction fault large enough to ensure that the effects of seismic and postseismic slip on the patches die out before reaching the boundaries of the friction region, so that the edges of the friction region move with the long-term slip rate consistent with the imposed rate outside. Table 1 Parameters of our simulations. Full size table Data availability The numerical data that support the findings presented and that have been used to produce the figures of this study are available from the corresponding authors upon request. How to cite this article: Lui, S. K. Y. & Lapusta, N. Repeating microearthquake sequences interact predominantly through postseismic slip. Nat. Commun. 7 , 13020 doi: 10.1038/ncomms13020 (2016).